Maintenance of neurotransmitter identity by Hox proteins through a homeostatic mechanism 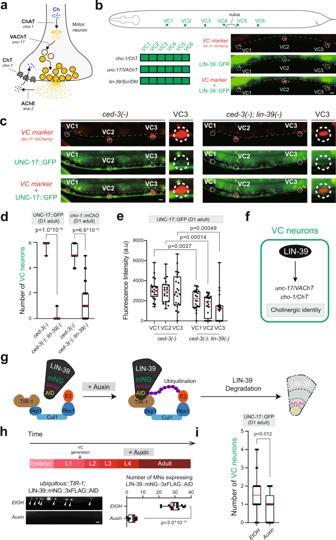Fig. 1: The Hox genelin-39 (Scr/Dfd/Hox4-5)is required to maintain the cholinergic identity of VC motor neurons. aPresynaptic bouton of a cholinergic motor neuron. Acetylcholine (ACh) pathway genes:cha-1/ChAT: Choline Acetyltransferase,unc-17/VAChT: Vesicular Acetylcholine Transporter,cho-1/ChT: Choline Transporter,ace-2/AChE: Acetylcholinesterase. Schematic adapted from Kratsios, P., et al., Coordinated regulation of cholinergic motor neuron traits through a conserved terminal selector gene.Nat. Neurosci. 15(2), 205–214 (2012).bCell body position of VC neurons in adultC. elegans. Bottom left: Co-expression ofcho-1, unc-17andlin-39in VC motor neurons. Bottom right: Representative image of a fosmid-basedlin-39reporter (LIN-39::GFP) and a VC-specific marker (lin-11::mCherry). GFP andmCherryco-localization occurs in all VC neurons; VC1-3 neurons are shown.cRepresentative images of UNC-17::GFP co-expressed withlin-11::mCherryinced-3(n1286) single andced-3 (n1286); lin-39(n1760) double mutants (day 1 adults). Inset shows VC3. Dashed circles: cell body positions. Dashed white lines: intestinal boundary; intestine is autofluorescent in the green channel.dQuantification ofunc-17andcho-1fosmid-based reporters inced-3(n1286) single andced-3 (n1286); lin-39(n1760) double mutants (day 1 adults).n= 17–23 animals.eFluorescence intensity quantification of UNC-17::GFP in VC1-3 inced-3(n1286) single andced-3 (n1286); lin-39(n1760) double mutants. See Material and Methods for details (a.u., arbitrary units).n= 22 animals.fSummary of LIN-39 function in VC MNs.gThe auxin-inducible protein degradation system. Skp1, Cul1, Rbx1, E2: components of E3 ligase complex. Worms express ubiquitously TIR1, a plant-specific substrate-recognizing subunit of the E3 ligase complex. With auxin, TIR1 binds to AID, leading to proteasomal degradation of LIN-39::mNG::3xFLAG::AID.hLIN-39::mNG::3xFLAG::AID depletion upon auxin. Representative images showing LIN-39::mNG::3xFLAG::AID expression in MNs upon auxin or EtOH treatment; quantifications on the right.n= 14 animals.iQuantification of the number of VC neurons expressing UNC-17::GFP upon auxin or EtOH treatment.n= 24 animals. For quantification ind,e,handi, box and whisker plots were used with the presentation of all data points. Box boundaries indicate the 25th and 75th percentile. The limits indicate minima and maxima values, whereas center values (mean) are highlighted in red. An unpairedt-test (two-sided) with Welch’s correction was performed. Source data are provided as a Source data file. Scale bars: 5 μm. Hox transcription factors play fundamental roles during early patterning, but they are also expressed continuously, from embryonic stages through adulthood, in the nervous system. However, the functional significance of their sustained expression remains unclear. In C. elegans motor neurons (MNs), we find that LIN-39 (Scr/Dfd/Hox4-5) is continuously required during post-embryonic life to maintain neurotransmitter identity, a core element of neuronal function. LIN-39 acts directly to co-regulate genes that define cholinergic identity (e.g., unc-17/VAChT, cho-1/ChT ). We further show that LIN-39, MAB-5 (Antp/Hox6-8) and the transcription factor UNC-3 (Collier/Ebf) operate in a positive feedforward loop to ensure continuous and robust expression of cholinergic identity genes. Finally, we identify a two-component design principle for homeostatic control of Hox gene expression in adult MNs: Hox transcriptional autoregulation is counterbalanced by negative UNC-3 feedback. These findings uncover a noncanonical role for Hox proteins during post-embryonic life, critically broadening their functional repertoire from early patterning to the control of neurotransmitter identity. Information flow in the nervous system critically relies on the ability of distinct neuron types to synthesize and package into synaptic vesicles specific chemical substances, known as neurotransmitters (NTs). Hence, a core functional feature of each neuron type is its NT identity, defined by the co-expression of genes encoding proteins necessary for the synthesis, packaging, and breakdown of a particular NT. Although rare instances of NT identity switching have been described in the nervous system [1] , [2] , it is generally accepted that individual neuron types acquire a specific NT identity during development and maintain it throughout life. In the case of cholinergic neurons, the enzyme choline acetyltransferase (ChAT) synthesizes acetylcholine (ACh) from its precursor choline, the vesicular ACh transporter (VAChT) packages ACh into synaptic vesicles, and the enzyme acetylcholinesterase (AChE) breaks down ACh upon its release into choline. The choline transporter (ChT) reuptakes choline back into the cholinergic neuron (Fig. 1a ) [3] . Co-expression of all these proteins throughout the life of a cholinergic neuron ensures the continuation of ACh biosynthesis, and thereby the communication of cholinergic neurons with their post-synaptic targets. Importantly, reduced expression of ACh pathway proteins has been associated with multiple neurological disorders [4] , [5] , [6] . Despite the widespread use of ACh in every nervous system [7] , [8] , how the co-expression of ACh pathway proteins is controlled over time, from development through adulthood, is poorly understood. A handful of studies in C. elegans and mice identified LIM and POU homeodomain transcription factors as necessary during development for ACh pathway gene expression in various types of cholinergic neurons [9] , [10] , [11] , [12] . However, the mechanisms that maintain the expression of ACh pathway genes during post-embryonic life are largely unknown. Fig. 1: The Hox gene lin-39 (Scr/Dfd/Hox4-5) is required to maintain the cholinergic identity of VC motor neurons. a Presynaptic bouton of a cholinergic motor neuron. Acetylcholine (ACh) pathway genes: cha-1 / ChAT : Choline Acetyltransferase, unc-17 / VAChT : Vesicular Acetylcholine Transporter, cho-1 / ChT : Choline Transporter, ace-2 / AChE : Acetylcholinesterase. Schematic adapted from Kratsios, P., et al., Coordinated regulation of cholinergic motor neuron traits through a conserved terminal selector gene. Nat. Neurosci . 15(2), 205–214 (2012). b Cell body position of VC neurons in adult C. elegans . Bottom left: Co-expression of cho-1, unc-17 and lin-39 in VC motor neurons. Bottom right: Representative image of a fosmid-based lin-39 reporter (LIN-39::GFP) and a VC-specific marker ( lin-11::mCherry ). GFP and mCherry co-localization occurs in all VC neurons; VC1-3 neurons are shown. c Representative images of UNC-17::GFP co-expressed with lin-11::mCherry in ced-3 ( n1286 ) single and ced-3 (n1286); lin-39 ( n1760 ) double mutants (day 1 adults). Inset shows VC3. Dashed circles: cell body positions. Dashed white lines: intestinal boundary; intestine is autofluorescent in the green channel. d Quantification of unc-17 and cho-1 fosmid-based reporters in ced-3 ( n1286 ) single and ced-3 (n1286); lin-39 ( n1760 ) double mutants (day 1 adults). n = 17–23 animals. e Fluorescence intensity quantification of UNC-17::GFP in VC1-3 in ced-3 ( n1286 ) single and ced-3 (n1286); lin-39 ( n1760 ) double mutants. See Material and Methods for details (a.u., arbitrary units). n = 22 animals. f Summary of LIN-39 function in VC MNs. g The auxin-inducible protein degradation system. Skp1, Cul1, Rbx1, E2: components of E3 ligase complex. Worms express ubiquitously TIR1, a plant-specific substrate-recognizing subunit of the E3 ligase complex. With auxin, TIR1 binds to AID, leading to proteasomal degradation of LIN-39::mNG::3xFLAG::AID. h LIN-39::mNG::3xFLAG::AID depletion upon auxin. Representative images showing LIN-39::mNG::3xFLAG::AID expression in MNs upon auxin or EtOH treatment; quantifications on the right. n = 14 animals. i Quantification of the number of VC neurons expressing UNC-17::GFP upon auxin or EtOH treatment. n = 24 animals. For quantification in d , e , h and i , box and whisker plots were used with the presentation of all data points. Box boundaries indicate the 25th and 75th percentile. The limits indicate minima and maxima values, whereas center values (mean) are highlighted in red. An unpaired t -test (two-sided) with Welch’s correction was performed. Source data are provided as a Source data file. Scale bars: 5 μm. Full size image Motor neurons (MNs) in the spinal cord of vertebrates and the ventral nerve cord of many invertebrates use ACh to communicate with their muscle targets. The nematode C. elegans contains six different classes (types) of MNs within its ventral nerve cord that are cholinergic [13] . Five classes (DA, DB, VA, VB, AS) control locomotion and are sex-shared (found in C. elegans males and hermaphrodites), whereas one class (VC) controls egg-laying and is found only in hermaphrodites. Each MN class contains several members (DA = 9 neurons, DB = 7, VA = 12, VB = 11, AS = 11, VC = 6) that intermingle along the nerve cord. The cholinergic identity of these MNs is defined by the expression of unc-17 (VAChT), cha-1 (ChAT), ace-2 (AChE), and cho-1 (ChT) (Fig. 1a ) [14] , [15] . The rapid life cycle of C. elegans (~3 days from embryo to adult), the established methods to inactivate transcription factor activity in the adult, and the availability of reporter animals for all ACh pathway genes offer a unique opportunity to probe in vivo, and with single-cell resolution, the molecular mechanisms that maintain cholinergic identity during post-embryonic life. Members of the HOX family of homeodomain transcription factors play fundamental roles during early development in anterior–posterior patterning and body plan formation [16] , [17] . Seminal studies in worms, flies, zebrafish, and mice have also established critical roles for Hox genes during the early development of the nervous system [18] , [19] , [20] , [21] , [22] . For example, Hox gene inactivation can affect the specification and/or survival of neuronal progenitors, as well as the differentiation, survival, migration, and/or connectivity of young post-mitotic neurons [18] , [19] , [20] , [21] , [22] . The focus on early development, however, combined with a lack of temporally controlled gene inactivation approaches that bypass early Hox pleiotropies (e.g., lethality, effects on neural progenitors) has resulted in an incomplete understanding of Hox gene functions in the nervous system. Emerging evidence in C. elegans, Drosophila , mice, and humans shows that Hox genes are expressed continuously, from development throughout adulthood, in certain neuron types [23] , [24] , [25] , [26] , [27] , [28] , [29] . However, the functional significance of sustained Hox gene expression in adult post-mitotic neurons remains unknown. Individual neuron types acquire their NT identity during development and maintain it throughout life. Previous work in C. elegans showed that the Hox gene lin-39 (Scr/Dfd/Hox4-5) is required for the production of serotonergic neurons in males and egg-laying (VC class) motor neurons in hermaphrodites [30] , [31] , [32] , [33] , [34] , but whether lin-39 acts in post-mitotic neurons to regulate NT identity genes was not tested. Hence, the role of Hox proteins in the control of NT identity remains unclear. Here, we show that LIN-39 is continuously required to maintain the expression of ACh pathway genes in cholinergic MNs, thereby securing their NT identity and function. In MNs that control locomotion, LIN-39 cooperates with another Hox protein MAB-5 (Antp/Hox6-8), and the transcription factor UNC-3 (Collier/Ebf) to directly activate the expression of ACh pathway genes. Moreover, LIN-39 and MAB-5 also regulate the expression levels of unc-3 , thereby generating a positive feedforward loop that ensures the robustness of ACh pathway gene expression throughout life. Importantly, we find that Hox gene expression is under homeostatic control and propose a two-component design principle that maintains optimal levels of Hox gene expression in MNs over time: Hox transcriptional autoregulation (component 1) is counterbalanced by negative UNC-3 feedback (component 2). Because Hox genes are expressed in the adult nervous system of invertebrate and vertebrate animals, their functional role in the maintenance of NT identity may be deeply conserved. The Hox gene lin-39 maintains the identity of motor neurons necessary for egg laying We initially focused on the hermaphrodite-specific VC MNs, for which regulators of their cholinergic identity remain unknown. The Hox gene lin-39 ( Scr/Dfd/Hox4-5 ) is continuously expressed in VC neurons, from the time they are born (larval stage 1, L1) until adulthood (Fig. 1b ) (Supplementary Fig. 1 ) [35] . However, animals carrying strong loss-of-function alleles for lin-39 lack VC neurons ( lin-39 controls VC survival) [31] , [33] , preventing us from testing its role in the regulation of VC cholinergic identity determinants unc-17/VAChT and cho-1/ChT (Supplementary Fig. 1 ) [15] . To bypass this, we generated double mutant animals for lin-39 and ced-3 (VC cell death depends on ced-3 caspase activity) [31] , [33] , and indeed observed that VC neurons are normally generated in these animals (Fig. 1c , Supplementary Fig. 1d, e ). Compared to controls, the number of VC neurons expressing unc-17 and cho-1 reporters was significantly reduced in lin-39(n1760); ced-3(n1286) double mutants in the adult (day 1) stage (Fig. 1c, d ). Subsequent fluorescence intensity analysis with higher resolution revealed that expression of the cholinergic marker unc-17::gfp is significantly reduced, but not completely eliminated (Fig. 1e ). For the unc-17 and cho-1 expression analysis, we used fosmid (~30 kb-long genomic clone)-based reporters, which despite their multicopy nature (overexpression), tend to faithfully recapitulate endogenous gene expression patterns [15] . Altogether, these findings suggest that, during larval development, lin-39 controls the expression of VC cholinergic identity determinants (Fig. 1f ). The sustained expression of lin-39 in VC MNs during adulthood raises the question of whether it is continuously required to maintain cholinergic identity. Because the lin-39(n1760) allele removes gene activity starting in early development, we used a previously validated lin-39::mNG::3xFLAG::AID allele that codes for a LIN-39 protein fused to mNG::3xFLAG (serves as an endogenous reporter) and auxin-inducible degron (AID) (enables LIN-39 depletion in a temporally-controlled manner) [36] , [37] (Fig. 1g ). We initiated auxin treatment at the last larval stage (L4) and maintained animals on auxin until the first day of adulthood (Fig. 1h ). This led to efficient LIN-39 depletion in VC neurons and other nerve cord MNs that normally express lin-39 (Fig. 1h ). In day 1 adults, although we observed a hypomorphic effect on unc-17 expression in the control group (ethanol [EtOH] treatment), we did witness a statistically significant decrease in the number of VC neurons expressing the unc-17 reporter in animals treated with auxin (Fig. 1i ). This indicates that lin-39 is required to maintain the expression of unc-17/VAChT at later life stages. Lastly, we examined two additional markers of VC terminal differentiation, ida-1 (ortholog of human protein tyrosine phosphatase receptor type N [PTPRN]) [38] and glr-5 (ortholog of human glutamate ionotropic receptor GRIK1) [39] . We found that lin-39 is continuously required to maintain ida-1 and glr-5 expression during late larval and adult stages (Supplementary Fig. 1d–f ). In conclusion, lin-39 , in addition to promoting VC survival during the L1 stage, is continuously required at later stages of life to control cholinergic identity gene expression (e.g., unc-17 ) and other features ( ida-1, glr-5 ) of VC terminal differentiation (Fig. 1f ). lin-39 controls the identity of motor neurons necessary for locomotion Prompted by our findings in MNs that control egg-laying, we next asked whether the control of NT identity by lin-39 extends to MNs that control locomotion. Using the endogenous lin-39::mNG::3xFLAG::AID reporter allele, we found lin-39 to be continuously expressed, from development to adulthood, in 28 of the 39 cholinergic MNs necessary for locomotion (Fig. 2a ) (Supplementary Fig. 1b ) [35] . These neurons survive in animals carrying the strong loss-of-function lin-39 allele (n1760) used in Fig. 1 [40] , enabling assessment of putative lin-39 effects on their cholinergic identity. Indeed, we found a significant decrease in the number of MNs expressing cho-1/ChT at L4 (Fig. 2b, c ). We obtained similar results for two additional cholinergic identity markers using an endogenous reporter for unc-17 (unc-17::mKate) and a fosmid-based reporter for ace-2/AChE (Fig. 2d, e ), suggesting lin-39 co-regulates the expression of several ACh pathway genes in MNs necessary for locomotion. The observed reduction in ACh pathway gene expression may account for the previously described locomotion defects of lin-39 mutant animals [36] . Fig. 2: The Hox gene lin-39 (Scr/Dfd/Hox4-5) controls the cholinergic identity of motor neurons necessary for locomotion. a Schematic of a C. elegans hermaphrodite showing the cell bodies of MNs that control locomotion (red) and egg-laying (green). Expression profile of cho-1, unc-17 , and lin-39 is summarized in the color-filled table. b Representative images of a cho-1 fosmid-based reporter in WT and lin-39(n1760) mutant animals (L4 stage). Motor neurons that control locomotion (e.g., DA, DB, VA, VB) express cho-1 at L4. VC motor neurons mature later (day 1 adult) and do not express cho-1 at L4. The identity of individual motor neurons is annotated. White arrowheads indicate MN nuclei because the cho-1 reporter is localized to the nucleus (H2B). mChOpti signal is shown in white for better contrast. Left image: anterior to the vulva, Right image: posterior to the vulva. c Quantification of the number of motor neurons expressing cho-1 in panel ( b ). The motor neurons that consistently lose cho-1 expression in lin-39(n1760) mutants are VA5, VB6, AS6, VA7, and VB8. n = 22 animals. d and e Quantification of the number of sex-shared motor neurons expressing unc-17 (endogenous reporter ot907 [UNC-17::mKate]) and ace-2 (fosmid-based reporter otEx4432 [ ace-2::GFP] ) in WT and lin-39(n1760) mutant hermaphrodites at L4. n = 19-25 animals. f and g Auxin treatment was initiated at L4 and images were scored at young adult stage (Day 1). Quantification of the number of sex-shared motor neurons expressing UNC-17::GFP upon auxin or EtOH treatment. n = 24 animals. For quantifications in c – f , box and whisker plots were used with the presentation of all data points. Unpaired t -test (two-sided) with Welch’s correction was performed and p -values were annotated. Box boundaries indicate the 25th and 75th percentile. The limits indicate minima and maxima values, whereas center values (mean) are highlighted in red. h Schematic summarizing our findings in MNs that control locomotion. Source data are provided as a Source data file. Scale bars: 5 μm. Full size image Due to its maintenance role in egg-laying MNs (Fig. 1g–i ), we next asked whether lin-39 is also required to maintain in the adult the cholinergic identity of MNs critical for locomotion. Again, we found that depletion of LIN-39 specifically during late larval and adult stages resulted in a decrease in the number of MNs expressing unc-17/ChAT (Fig. 2f, g ), strongly suggesting a continuous LIN-39 requirement in these neurons. lin-39 cooperates with mab-5 and unc-3 to control the identity of motor neurons Compared to the strong effects observed in VC MNs (Fig. 1d ), we observed modest effects on ACh pathway gene expression upon lin-39 loss in MNs that control locomotion (Fig. 2c–f ), suggesting additional factors partially compensate for lin-39 in these neurons (Fig. 2h ). To identify them, we followed a candidate approach. First, we reasoned that mab-5 ( Antp, Hox6-8 ), another Hox gene with continuous expression in a subset of lin-39 -expressing MNs (Fig. 3a ) (Supplementary Fig. 2 ) [26] , may work together with lin-39 to control NT identity features. To test this, we generated double lin-39(n1760); mab-5(e1239) mutant animals. All MNs that control locomotion are normally generated in this mutant [40] . However, we observed a decrease in the number of MNs expressing the cholinergic marker unc-17/VAChT in double lin-39(n1760); mab-5(e1239) mutants compared to single lin-39(n1760) mutant animals (Fig. 3d ). Moreover, the residual expression of unc-17/VAChT in MNs of lin-39; mab-5 double mutants suggests that, besides MAB-5, additional regulatory factors must cooperate with LIN-39. The transcription factor UNC-3, a member of the Collier/Olf/Ebf (COE) family, is selectively expressed in MNs that control locomotion (Fig. 3a ) and is the only factor previously known to control their cholinergic identity [14] . Hence, if unc-3 compensates for the combined loss of lin-39 and mab-5 , we would predict stronger effects on ACh pathway gene expression in MNs of triple mutant unc-3(n3435); lin-39(n1760); mab-5(e1239) animals than in single unc-3 or double lin-39; mab-5 mutants. Indeed, this was the case for cho-1/ChT and ace-2/AChE expression (Fig. 3b, c, e ). Because animals carrying the strong loss-of-function unc-3 allele (n3435) [41] display a striking reduction in the number of MNs expressing unc-17/VAChT (UNC-3 is absolutely required for unc-17/VAChT ) (Fig. 3d ), we used a hypomorphic (weaker loss-of-function) unc-3 allele (ot837) [36] to test the notion of cooperation. Indeed, we observed stronger effects on unc-17/VAChT expression in unc-3 (ot837); lin-39(n1760); mab-5(e1239) compared to unc-3 (ot837), and double lin-39; mab-5 mutants (Fig. 3d ). We extended the analysis of the hypomorphic unc-3 allele (ot837) to cho-1/ChT , and again observed stronger effects in triple mutant animals (Fig. 3b, c, e ). Although the magnitude of the observed effects differs in Hox and unc-3 mutants, this genetic analysis suggests that lin-39, mab-5 , and unc-3 synergize to control the expression of several ACh pathway genes in MNs necessary for C. elegans locomotion (Fig. 3f ). Fig. 3: lin-39 cooperates with mab-5 (Antp, Hox6-8) and unc-3 (Collier/Ebf) to control cholinergic motor neuron identity. a Schematic of a C. elegans hermaphrodite showing the cell bodies of MNs that control locomotion (red) and egg-laying (green). The expression profile of cho-1, unc-17, unc-3, lin-39, and mab-5 is illustrated in the color-filled table below. b Representative images of a cho-1 fosmid-based reporter at L4 in the genetic background of WT, lin-39(-), mab-5(-), lin-39(-) mab-5(-), unc-3(-), unc-3(-); lin-39(-), unc-3(-); lin-39(-) mab-5(-), unc-3(hypo), and unc-3(hypo); lin-39(-) mab-5(-) . Strong-loss-of-function (null) alleles of lin-39(n1760), mab-5(e1239), and unc-3(n3435) are annotated as (-) and the hypomorphic unc-3 allele ot837 [unc-3::mNG::AID] as (hypo ). The identity of individual motor neurons is annotated. White arrowheads indicate MN nuclei because the cho-1 reporter is localized to the nucleus (H2B). mChOpti signal is shown in white for better contrast. Left image: anterior to the vulva, Right image: posterior to the vulva. c Quantification of the number of motor neurons expressing cho-1 in panel ( b ). n = 16–23 animals. d and e Quantification of the number of motor neurons (that control locomotion) expressing unc-17 (endogenous reporter ot907 [UNC-17::mKate]) and ace-2 (fosmid-based reporter otEx4432 [ ace-2::GFP ]) in multiple genetic backgrounds at L4 stage. n = 16–25 animals. For quantifications in c – e , box and whisker plots were used with the presentation of all data points. Unpaired t -test (two-sided) with Welch’s correction was performed and p -values were annotated. Box boundaries indicate the 25th and 75th percentile. The limits indicate minima and maxima values, whereas center values (mean) are highlighted in red. f Schematic summarizing our findings in cholinergic motor neurons that control locomotion. Source data are provided as a Source data file. Scale bar: 5 μm. Full size image LIN-39 and UNC-3 act through distinct binding sites to activate ACh pathway gene expression Interrogation of available ChIP-Seq datasets provided biochemical evidence of UNC-3 binding to the cis -regulatory regions of ACh pathway genes ( unc-17/VAChT, cho-1/ChT, ace-2/AChE ) (Fig. 4a, d ) (Supplementary Fig. 3 ) [42] . These bound regions contain cognate sites for UNC-3, and their previous mutational analysis strongly suggested UNC-3 acts directly to activate ACh pathway gene expression in cholinergic MNs [14] . Next, we examined available ChIP-Seq datasets for LIN-39 and MAB-5 [43] , and witnessed coincident binding of LIN-39, MAB-5, and UNC-3 at cis -regulatory regions of unc-17/VAChT, cho-1/ChT , and ace-2/AChE (Fig. 4a, d , Supplementary Fig. 3 ). We hypothesized that these co-bound regions (putative enhancers) are sufficient to drive reporter ( yfp ) gene expression in MNs. Indeed, a 280bp-long fragment of the cho-1 cis -regulatory region, as well as two fragments (1000 and 125 bp) of the unc-17 region, are sufficient to drive yfp expression in MNs (Fig. 4a, b, d–f ). The yfp expression driven by these putative enhancer regions ( cho-1_280bp, unc-17_1000bp, unc-17_125bp ) is unc-3 - and Hox-dependent (Fig. 4b, c, e, f ), as evidenced by a reduction in the number of MNs expressing the yfp reporter. Similar to our observations with an endogenous reporter for unc-17 and a fosmid-based reporter for cho-1 (Fig. 3c, d ), we corroborated the notion of synergy between UNC-3 and Hox by using the hypomorphic unc-3 allele (ot837) . Stronger effects were observed in unc-3 (ot837); lin-39; mab-5 triple mutants compared to unc-3(ot837) single or lin-39; mab-5 double mutant animals (Fig. 4c, e, f ). Altogether, our enhancer analysis in unc-3 and Hox mutants identified specific cis -regulatory regions that require both UNC-3 and Hox (LIN-39, MAB-5) input to drive unc-17/VAChT and cho-1/ChT expression in cholinergic MNs. Fig. 4: LIN-39 and UNC-3 act directly to activate the expression of ACh pathway genes. a Gene locus of cho-1 with ChIP-seq tracks for UNC-3, LIN-39, and MAB-5. Molecular nature of cho-1 reporter gene cho-1::mChOpti and cho-1_280 bp::YFP is shown. Total number of MNs expressing each reporter is indicated in the format of mean ± standard derivation (SD). Within a 280 bp cis -regulatory region (gray dashed line), an UNC-3 site and a predicted LIN-39 site are highlighted in red and blue, respectively. MAB-5 binding sites are not shown because they are not well-defined. b Representative images of cho-1_280bp::YFP expression at L4 in WT, unc-3(n3435), lin-39(n1760) mab-5(e1239), unc-3(hypo), and unc-3(hypo); lin-39(n1760); mab-5(e1239) animals. Arrowheads indicate MN nuclei because cho-1_280bp::YFP has a nuclear localization signal (NLS). YFP signal is shown in white for better contrast. Dashed white lines indicate the boundary of the intestine, which is auto-fluorescent in the green channel. c Quantification of the number of motor neurons expressing cho-1 reporter in panel ( b ). n = 18–27 animals. d . Gene locus of unc-17 with ChIP-seq tracks for UNC-3, LIN-39, and MAB-5. Expression in motor neurons is quantified for unc-17 reporter genes ( unc-17_1kb::YFP and unc-17_125bp::YFP), as well as its mutated version with LIN-39 site deletions. Within a 125 bp cis -regulatory region framed by the gray dashed line, a UNC-3 site and 4 predicted LIN-39 sites are highlighted in red and blue, respectively. e and f Quantification of the number of motor neurons at L4 expressing the unc-17_1kb::YFP ( e ) and unc-17_125bp::YFP ( f ) reporters in WT, unc-3(n3435), lin-39(n1760); mab-5(e1239), unc-3(n3435), lin-39(n1760); mab-5(e1239), unc-3(hypo), and unc-3(hypo); lin-39(n1760); mab-5(e1239) animals. For all quantifications, box and whisker plots were used with the presentation of all data points. Box boundaries indicate the 25th and 75th percentile. The limits indicate minima and maxima values, whereas center values (mean) are highlighted in red. Unpaired t -test (two-sided) with Welch’s correction was performed and p-values were annotated. n = 15–26 animals. g Schematic of unc-17 regulation by UNC-3, LIN-39, and MAB-5. Red and blue rectangles indicate the binding sites of UNC-3 and LIN-39, respectively. Source data are provided as a Source data file. Scale bar: 5 μm. Full size image Within the cho-1_280bp and unc-17_125bp enhancer regions, a single UNC-3 binding site (COE motif) is necessary for reporter gene expression in MNs (Fig. 4a, d ) [14] . We bioinformatically searched for the presence of consensus LIN-39-binding sites (GATTGATG), which, unlike MAB-5 sites, are well-defined in C. elegans [43] . We found a single LIN-39 binding site 60 bp upstream of the UNC-3 site in the cho-1_280bp region (Fig. 4a ) and four LIN-39 sites flanking the UNC-3 binding site in the unc-17_125bp region (Fig. 4d ). We tested the functional importance of the 4 LIN-39 sites by simultaneously deleting them in the context of transgenic reporter ( unc-17_125bp::yfp) animals, and found a dramatic decrease in yfp expression in MNs (Fig. 4d ). Altogether, this analysis combined with the ChIP-Seq results provide strong evidence that LIN-39 and UNC-3 bind directly to the cis -regulatory region of ACh pathway genes, and recognize distinct binding sites (Fig. 4g ). A positive feed-forward loop (FFL) for the control of cholinergic motor neuron identity Our findings suggest that Hox proteins LIN-39 and MAB-5, like UNC-3, directly control the expression of ACh pathway genes in MNs. However, LIN-39 and MAB-5 also bind extensively on the cis -regulatory region of unc-3 (Fig. 5a ), suggesting they directly regulate its expression as well. Indeed, expression of an endogenous gfp reporter for unc-3 (UNC-3::GFP protein fusion) is significantly reduced in MNs of lin-39 single mutants, and this effect is exacerbated in lin-39; mab-5 double mutants (Fig. 5b, c ). The number of MNs that express UNC-3::GFP is lower in lin-39 and lin-39; mab-5 animals (left graph in Fig. 5c ). Compared to WT, we also observed a striking reduction in UNC-3::GFP fluorescence intensity in MNs of Hox mutant animals (34% reduction in lin-39 and 43% in lin-39; mab-5 ) (middle graph in Fig. 5c ), suggesting lin-39 and mab-5 are required for normal levels of UNC-3 expression. Fig. 5: LIN-39 and MAB-5 control unc-3 expression levels. a ChIP-seq tracks for LIN-39 and MAB-5 on unc-3 locus. Molecular nature of endogenous unc-3 reporters (UNC-3::GFP and UNC-3::GFP LIN-39 site MUT ) and transgenic unc-3 reporters (unc-3_223bp::mChe, unc-3_ΔExon3-11_mChe , unc-3_ΔExon7-11_mChe) . b Representative images of L4 animals carrying the endogenous unc-3::gfp reporter in WT, lin-39(n1760) , and lin-39(n1760); mab-5(e1239) backgrounds. c Quantification of MN number (left graph, n = 19–22 animals) or fluorescence intensity (middle graph, n = 595 neurons) of UNC-3::GFP in WT , lin-39(n1760), and lin-39(n1760); mab-5(e1239) backgrounds. Right graph: Quantification of fluorescent GFP intensity in MNs of animals carrying the UNC-3::G FP and UNC-3::GFP LIN-39 site MUT endogenous reporters. n = 682 neurons. d Quantification of the number of unc-3 mRNA fluorescence aggregates in individual cholinergic MNs. Single-molecule mRNA FISH for unc-3 was performed in WT and lin-39(n1760); mab-5(e1239) animals at L1. For all quantifications, box and whisker plots were used; all data points shown. Unpaired t -test with Welch’s correction was performed and p -values were annotated. n = 22 animals. Representative images of DB5, DA5, DB7, and DA7 neurons. WT (colored red) versus mutant (in blue) for quantification. Magenta: signal from Quasar 670 probe for unc-3 mRNA, Green: unc-17::gfp reporter for cholinergic motor neurons. e Representative images of unc-3_223bp::mChe expression in L4 hermaphrodites in WT, lin-39(n1760) , and lin-39(n1760); mab-5(e1239) . f and g Quantification of MN numbers ( f , n = 13–17 animals) or fluorescence intensity ( g , n = 176 neurons) of unc-3_223bp::mChe in panel ( e ). For fluorescence intensity quantifications, single neurons expressing the mCherry reporters are plotted as individual data points. n > 600. In panel g , n > 200 neurons. h and i Quantification of the number of MNs expressing the unc-3_ΔExon3-11_mChe ( h ), and unc-3_ΔExon7-11_mChe ( i ) in WT and lin-39(n1760); mab-5(e1239) mutant animals. n = 10 animals. For all quantifications, box and whisker plots were used; all data points were presented. Box boundaries indicate the 25th and 75th percentile. The limits indicate minima and maxima values, whereas center values (mean) are highlighted in red. Unpaired t -test (two-sided) with Welch’s correction was performed. j Schematic model of a coherent feed-forward loop (FFL) for the control of cholinergic identity. Source data are provided as a Source data file. Scale bars: 5 μm. Full size image The binding of LIN-39 and MAB-5 on the unc-3 locus strongly suggests these Hox proteins control unc-3 expression by acting at the level of transcription. Four lines of evidence support this possibility. First, CRISPR/Cas9-mediated mutation of a predicted LIN-39 binding site in the context of the endogenous unc-3::gfp reporter (UNC-3::GFP LIN-39 site MUT ) resulted in decreased expression in MNs (right graph in Fig. 5a, c ). Second, we quantified endogenous unc-3 mRNA levels with single-cell resolution using RNA fluorescent in situ hybridization (RNA FISH) [44] . Compared to wild-type animals, we observed a consistent decrease of unc-3 mRNA levels in cholinergic MNs of lin-39; mab-5 mutants (Fig. 5d ). Similar results were obtained with RT-PCR in animals carrying a hypomorphic lin-39 allele (Supplementary Fig. 4 ). Third, a small 223 bp-long cis -regulatory element upstream of the first unc-3 exon is sufficient to drive reporter gene ( mCherry ) expression in wild-type MNs (Fig. 5a, e ). When we quantified the number of MNs expressing this reporter, as well as its fluorescence intensity, we observed statistically significant differences in Hox mutant animals (Fig. 5f, g ). Like our observations with the UNC-3::GFP fusion (Fig. 5b, c ), we observed a 28% reduction in fluorescence intensity of the unc-3_223bp::mCherry reporter in lin-39 single mutants, which was exacerbated (34% reduction) in lin-39; mab-5 double mutants (Fig. 5g ). Lastly, we generated two fosmid-based reporters, in which we replaced two different parts of the unc-3 locus (exon 3–11 [ΔExon3–11], exon7–11 [ΔExon7–11]) with mCherry while leaving the upstream and downstream cis -regulatory elements intact (Fig. 5a ). In both cases, we found a significant reduction in the number of mCherry -expressing MNs in lin-39; mab-5 double mutant animals (Fig. 5h, i ). We note that unc-3 expression is not completely abolished in motor neurons of lin-39; mab-5 mutants (Fig. 5b–i ), indicating that there must be additional, yet-to-be-identified factors that activate unc-3 and compensate for the combined loss of lin-39 and mab-5 . Altogether, Hox proteins (LIN-39, MAB-5) act directly to activate the expression of ACh pathway genes in MNs (Hox → ACh genes, Figs. 3 and 4 ). Further, Hox proteins act at the level of transcription to control unc-3 , which also controls ACh genes (Hox → unc-3 → ACh genes), thereby generating a positive feed-forward loop (FFL) (Fig. 5j ). lin-39 and mab-5 maintain their expression through transcriptional autoregulation How is Hox gene expression maintained in adult MNs? Available ChIP-Seq data show LIN-39 binding at its own locus in vivo (Fig. 6a ), consistent with in vitro observations [45] . This raises the possibility of lin-39 maintaining its own expression in MNs through transcriptional autoregulation. To test this, we first determined which cis -regulatory elements of the lin-39 locus are sufficient to drive reporter ( TagRFP ) expression in MNs. A 6.2 kb element upstream of the lin-39 locus fused to TagRFP only shows low levels of expression in a small number of nerve cord MNs (~6) during larval stages (Fig. 6a ). This prompted us to study intronic elements. When intron 1 of lin-39 was fused to TagRFP , we detected robust TagRFP expression in ~23 nerve cord MNs, consistent with a previous study [45] . These lin-39 intron 1 ::TagRFP animals display continuous expression in both larval and adult MNs (Fig. 6a, b ), similar to animals carrying the endogenous lin-39 reporter allele ( lin-39::mNG::3xFLAG::AID ), enabling us to test the idea of transcriptional autoregulation. Indeed, the number of TagRFP -expressing MNs is significantly reduced in lin-39 homozygous mutants carrying a null allele ( n1760 ) (Fig. 6b ), suggesting lin-39 gene activity is necessary for its expression in MNs. Fig. 6: Transcriptional autoregulation of lin-39 in motor neurons. a ChIP-seq tracks for LIN-39 on lin-39 locus. Molecular nature of endogenous lin-39 reporters ( lin-39::mNG::3xFLAG::AID and lin-39::mNG::3xFLAG::AID sites1-11MUT ) and transgenic lin-39 reporters (lin-39_6.2kb::tagRFP , lin-39 intron1 ::tagRFP, lin-39_832bp::tagRFP , lin-39_776bp::tagRFP , 776bp_Δsite#1::tagRFP , 776bp_Δsite#9::tagRFP ). The mean value of MNs that express each reporter is indicated on the right. The precise location of the 11 predicted LIN-39 binding sites is shown, and their mutated version. b Representative images and quantification of the number of MNs expressing lin-39 intron1 ::tagRFP in WT and lin-39(n1760) mutants at L4. n = 21–30 animals. c Depletion of LIN-39::mNG::3xFLAG::AID upon auxin. Worms expressing the lin-39::mNG::3xFLAG::AID together with TIR protein in all neurons (driven by pan-neuronal promoter otti28 ) were grown on normal OP50 plates until L2 stage and then transferred to plates containing either auxin or EtOH (as control). Animals were imaged at L4. Quantification of LIN-39::mNG::3xFLAG::AID expression in motor neurons upon Auxin or EtOH treatment. n = 8–15 animals. d Representative images and quantification of the number of MNs expressing lin-39 intron1 ::tagRFP treated with EtOH or auxin. n = 26-28 animals. e and f Quantification (L4 stage) of the number of MNs expressing mNG ( e , n = 18–19 animals) or the fluorescence intensity ( f , n = 459 neurons) of mNG in animals carrying the lin-39::mNG::3xFLAG::AID and lin-39::mNG::3xFLAG::AID sites1-11MUT alleles. In panel f , single neurons expressing mNG are plotted as individual data points. n > 400 cells. a.u. arbitrary units. g Quantification of fluorescent intensity of cho-1::SL2::mChOpti::H2B expression in MNs of lin-39::mNG::3xFLAG::AID or lin-39::mNG::3xFLAG::AID sites1-11MUT animals (L4 stage). h Quantification of the number of MNs expressing the lin-39_776bp::tagRFP reporter (intact and mutated version with LIN-39 site#1 or #9 mutated). Two independent transgenic lines for each version of the reporter were used. n = 12–21 animals. For all quantifications, box and whisker plots were used; all data points were presented. Box boundaries indicate the 25th and 75th percentile. The limits indicate minima and maxima values, whereas center values (mean) are highlighted in red. Unpaired t -test (two-sided) with Welch’s correction was performed. n > 15 animals. i Schematic model of lin-39 transcriptional autoregulation. j Schematic model showing the autoregulation of lin-39 embedded at the top of a coherent FFL. Source data are provided as a Source data file. Scale bars: 5 μm. Full size image Because the lin-39 (n1760) allele removes gene activity starting in the early embryos, the above findings do not address whether LIN-39 is continuously required to maintain its expression at later stages. To test this, we again used the AID system and efficiently depleted LIN-39 protein levels during late larval stages (Fig. 6c ). Upon auxin administration, we found a significant reduction in the number of MNs expressing the lin-39 intron 1 ::TagRFP reporter (Fig. 6d ), suggesting lin-39 is continuously required to maintain its own expression. These findings pinpoint the entirety of intron 1 as a putative cis -regulatory region used by LIN-39 to directly control its own expression. Next, we generated transgenic reporter animals that split intron 1 into two fragments (832 and 776 bp). Animals carrying the 776 bp fragment ( lin-39 776bp ::TagRFP) revealed reporter gene expression in nerve cord MNs, but that was not the case for the 832 bp fragment (Fig. 6a ). Within the 776 bp fragment, we found 11 predicted LIN-39 binding sites (motifs) (Fig. 6a ), and employed CRISPR/Cas9 gene editing to simultaneously mutate all of them in the context of the endogenous lin-39::mNG::3xFLAG::AID reporter allele (SunyBiotech). This led not only to a decrease in the number of MNs expressing the endogenous lin-39::mNG::3xFLAG::AID sites 1-11 MUT reporter (Fig. 6e ) but also to a reduction of its expression levels (Fig. 6f ). These findings support a transcriptional autoregulation model where LIN-39 recognizes its cognate binding sites within intron 1 to regulate its expression in nerve cord MNs (Fig. 6i ). Importantly, we observed functional consequences when lin-39 autoregulation was selectively disrupted; the expression levels of cho-1/ChT in cholinergic MNs were significantly reduced in animals carrying the lin-39::mNG::3xFLAG::AID sites 1–11 MUT allele (Fig. 6g ). To investigate which of the 11 LIN-39 sites are functionally important, we mutated two sites with the highest bioinformatic prediction scores (sites #1 and #9 in Fig. 6a , see the “Methods” section). Mutation of either site in the context of lin-39 776bp ::TagRFP animals significantly decreased the number of TagRFP -expressing MNs (Fig. 6h ), indicating that these sites are necessary for autoregulation. Lastly, we asked whether the Hox gene mab-5 , like lin-39 , controls its own expression in MNs. Supporting this possibility, ChIP-Seq data show extensive MAB-5 binding at its own locus, and expression of a mab-5::gfp reporter is significantly reduced in MNs of mab-5 mutant animals (Supplementary Fig. 5 ). Altogether, these findings uncover a positive feedback mechanism (transcriptional autoregulation) required to maintain Hox gene expression in MNs (Fig. 6j ). UNC-3 (Collier/Ebf) prevents high levels of Hox gene ( lin-39 , mab-5 ) expression Low levels of LIN-39 lead to a failure to maintain ACh pathway gene expression at appropriate levels (Figs. 1 and 2 ), whereas high levels of LIN-39 in cholinergic MNs result in locomotion defects [36] . Hence, we hypothesized that the levels of lin-39 in cholinergic MNs must be tightly controlled to avoid detrimental effects on MN function (see the “Discussion” section). The findings described below suggest that tight control of Hox gene expression in MNs is achieved through a two-component mechanism, that is, Hox transcriptional autoregulation is counterbalanced by negative UNC-3 feedback. Because UNC-3 ChIP binding peaks are observed in lin-39 and mab-5 loci (Fig. 7a , Supplementary Fig. 6a ), we reasoned that UNC-3 acts directly to prevent high levels of Hox gene expression in cholinergic MNs. Multiple lines of evidence support this idea. First, the expression levels of the endogenous lin-39::mNG::3xFLAG::AID reporter are increased in MNs of unc-3 mutant animals (Fig. 7b, c ). Second, the lin-39 intron 1 ::TagRFP reporter showed increased TagRFP expression in MNs of unc-3 null (Fig. 7d, e ) and hypomorphic (Supplementary Fig. 7a ) mutants. Lastly, RNA FISH revealed increased levels of lin-39 mRNA molecules in individual MNs of unc-3 mutants (Fig. 7f ). Importantly, we extended this analysis to mab-5 , and obtained similar results; unc-3 gene activity is necessary to prevent high levels of mab-5 expression in MNs (Supplementary Fig. 6b, c ). Fig. 7: UNC-3 (Collier/Ebf) prevents high levels of lin-39 expression. a Gene locus of lin-39 with ChIP-seq tracks for UNC-3 and LIN-39. Molecular nature of lin-39 reporter gene lin-39::mNG::3xFLAG::AID and lin-39 intron1 ::tagRFP is shown. b and c Representative images ( b ) and quantifications ( c ) of the number of MNs ( n = 20 animals) expressing lin-39::mNG::3xFLAG::AID and the fluorescence intensity ( n = 660 neurons) in WT and unc-3(n3435) animals at L4. d and e Representative images ( d ) and quantifications ( e ) of the number ( n = 23 animals) and the fluorescence intensity ( n = 264 neurons) of MNs expressing lin-39 intron1 ::tagRFP in WT versus unc-3(n3435) animals at L4. In panels c and e , single neurons expressing the indicated reporter gene are evaluated for fluorescence intensity and plotted as individual data points in the graph. n > 600 neurons. a.u. arbitrary unit. f Quantification of the number of lin-39 mRNA fluorescence aggregates in individual cholinergic MNs. Single-molecule mRNA FISH for lin-39 ( using a Quasar 670 fluorescent probe) was performed in WT and unc-3(n3435) animals at L1 ( n = 20 animals). For all quantifications, box and whisker plots were used with the presentation of all data points. Box boundaries indicate the 25th and 75th percentile. The limits indicate minima and maxima values, whereas center values (mean) are highlighted in red. Unpaired t -test (two-sided) with Welch’s correction was performed and p -values were annotated. n > 20 animals. Representative images of DA3, DB4, DB7, and DA7 are shown. WT data is colored red versus mutant in blue for quantification. Images are shown in merged channels. Magenta: signal from Quasar 670 probe for lin-39 mRNA, Blue: DAPI for nuclei staining. g Schematic model of the gene regulatory network for maintenance of cholinergic identity in C. elegans motor neurons. Source data are provided as a Source data file. Scale bars: 5 μm. Full size image We next asked whether reducing UNC-3 levels by selectively disrupting the Hox input onto the unc-3 locus can affect the expression of cholinergic identity genes. For this, we used the UNC-3::GFP LIN-39 site MUT allele, in which we observed lower levels of UNC-3 expression in motor neurons (Fig. 5a–c ). We found that the expression levels of cholinergic identity genes ( unc-17/VAChT, cho-1/ChT ) are increased in motor neurons of animals carrying this allele (Supplementary Fig. 8 ), consistent with our model of low UNC-3 levels leading to a lack of efficient Hox gene repression (Fig. 7g ). Taken together, our findings uncover an intricate gene regulatory network for the maintenance of cholinergic identity in C. elegans MNs. This network contains a positive FFL, where Hox proteins (LIN-39 and MAB-5) not only activate the expression of ACh pathway genes but also control the expression of unc-3 , a critical regulator of cholinergic identity in MNs (Fig. 7g ). Moreover, the top level of this FFL, i.e., Hox, is under homeostatic control, ensuring that optimal levels of Hox gene expression are maintained in MNs. This is achieved through Hox transcriptional autoregulation counterbalanced by negative UNC-3 feedback (Fig. 7g ). Hox genes play fundamental roles in early patterning and body plan formation, but their functions in later stages of development and post-embryonic life remain largely unknown. 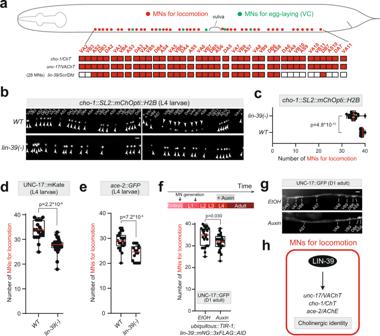Fig. 2: The Hox genelin-39 (Scr/Dfd/Hox4-5)controls the cholinergic identity of motor neurons necessary for locomotion. aSchematic of aC. eleganshermaphrodite showing the cell bodies of MNs that control locomotion (red) and egg-laying (green). Expression profile ofcho-1, unc-17, andlin-39is summarized in the color-filled table.bRepresentative images of acho-1fosmid-based reporter inWTandlin-39(n1760)mutant animals (L4 stage). Motor neurons that control locomotion (e.g., DA, DB, VA, VB) expresscho-1at L4. VC motor neurons mature later (day 1 adult) and do not expresscho-1at L4. The identity of individual motor neurons is annotated. White arrowheads indicate MN nuclei because thecho-1reporter is localized to the nucleus (H2B).mChOptisignal is shown in white for better contrast. Left image: anterior to the vulva, Right image: posterior to the vulva.cQuantification of the number of motor neurons expressingcho-1in panel (b). The motor neurons that consistently losecho-1expression inlin-39(n1760)mutants are VA5, VB6, AS6, VA7, and VB8.n= 22 animals.dandeQuantification of the number of sex-shared motor neurons expressingunc-17(endogenous reporterot907[UNC-17::mKate]) andace-2(fosmid-based reporterotEx4432[ace-2::GFP]) in WT andlin-39(n1760)mutant hermaphrodites at L4.n= 19-25 animals.fandgAuxin treatment was initiated at L4 and images were scored at young adult stage (Day 1). Quantification of the number of sex-shared motor neurons expressing UNC-17::GFP upon auxin or EtOH treatment.n= 24 animals. For quantifications inc–f, box and whisker plots were used with the presentation of all data points. Unpairedt-test (two-sided) with Welch’s correction was performed andp-values were annotated. Box boundaries indicate the 25th and 75th percentile. The limits indicate minima and maxima values, whereas center values (mean) are highlighted in red.hSchematic summarizing our findings in MNs that control locomotion. Source data are provided as a Source data file. Scale bars: 5 μm. In the context of the nervous system, Hox genes are known to control early events, such as specification, survival, and/or migration of progenitor cells and young post-mitotic neurons [18] , [19] , [20] , [21] , [22] . Here, we identify a critical role for Hox proteins during the later stages of nervous system development and post-embryonic life, critically extending their functional repertoire beyond early patterning. Using C. elegans nerve cord MNs as a model, we found that Hox gene activity is continuously required from development through adulthood for the control of NT identity, a core element of neuronal function. Moreover, Hox genes operate in a positive feedforward loop to safeguard the cholinergic identity of MNs: they not only control directly ACh pathway genes (e.g., unc-17/VAChT , cho-1/ChT ), but also the expression of unc-3 ( Collier/Ebf ), a master regulator of MN identity [14] . Lastly, we propose a homeostatic mechanism that maintains Hox gene expression in MNs at optimal levels, thereby ensuring the robust expression of cholinergic identity determinants throughout life. Hox genes lin-39 ( Scr/Dfd, Hox4-5 ) and mab-5 (Antp, Hox6-8) act as terminal selectors of cholinergic MN identity Transcription factors that are continuously expressed in individual neuron types and act directly to co-regulate the expression of NT pathway genes have been termed “terminal selectors” [46] , [47] , [48] . Terminal selectors have been described to date for various neuron types in C. elegans , flies, simple chordates, and mice, indicating the evolutionary conservation of terminal selector-based mechanisms for the control of NT identity [49] , [50] . The sustained expression of terminal selectors in specific neuron types suggests they are continuously required to maintain NT identity. However, a continuous requirement has been experimentally demonstrated only for a handful of terminal selectors to date [51] . Recent work in C. elegans , flies, and mice indicates that certain Hox genes are continuously expressed, from development through adulthood, in distinct neuron types [23] , [24] , [25] , [26] , [27] , [28] , [29] . Functional studies in peptidergic neurons in Drosophila , as well as hindbrain and spinal neurons in mice, showed that Hox proteins control early facets of neuronal development (e.g., specification, survival, migration, connectivity) [18] , [19] , [20] , [21] , [22] , [52] , but whether they function as terminal selectors remains unknown—in part due to a lack of temporally controlled studies for Hox gene inactivation later in life. Through constitutive (genetic null alleles) and post-embryonic (inducible protein depletion) approaches, we found that the Hox gene lin-39 is continuously required to maintain the cholinergic identity of C. elegans MNs. Biochemical (ChIP-Seq) and genetic evidence strongly suggest that LIN-39 and another Hox protein (MAB-5) act directly to co-regulate the expression of genes that encode integral components of the ACh biosynthetic pathway ( unc-17/VAChT , cho-1/ChT , ace-2/AChE ). Collectively, these findings reveal that Hox proteins can act as terminal selectors, uncovering a noncanonical role for these highly conserved transcription factors. Because Hox genes are expressed in various neuron types in C. elegans [29] , we surmise they may function as terminal selectors in other neurons as well. Supporting this notion, expression of a single marker of serotonergic identity ( tph-1 , tryptophan hydroxylase 1 [TPH1]) is affected in CP neurons of lin-39 mutant animals [53] , [54] . Similarly, expression of a dopaminergic identity marker ( cat-2 /tyrosine hydroxylase [TH]) is affected in tail sensory neurons of animals lacking activity of the posterior Hox gene egl-5 ( AbdB ) [55] . Future work is needed, however, to establish whether in those neurons LIN-39 and EGL-5 act as bona fide terminal selectors. 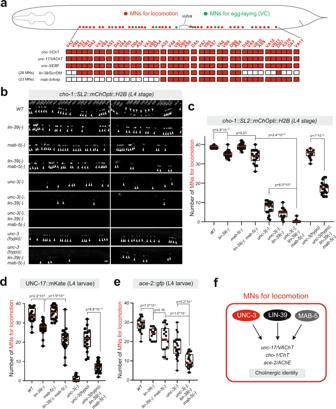Fig. 3:lin-39cooperates withmab-5 (Antp, Hox6-8)andunc-3 (Collier/Ebf)to control cholinergic motor neuron identity. aSchematic of aC. eleganshermaphrodite showing the cell bodies of MNs that control locomotion (red) and egg-laying (green). The expression profile ofcho-1, unc-17, unc-3, lin-39,andmab-5is illustrated in the color-filled table below.bRepresentative images of acho-1fosmid-based reporter at L4 in the genetic background ofWT, lin-39(-), mab-5(-), lin-39(-) mab-5(-), unc-3(-), unc-3(-); lin-39(-), unc-3(-); lin-39(-) mab-5(-), unc-3(hypo), and unc-3(hypo); lin-39(-) mab-5(-). Strong-loss-of-function (null) alleles oflin-39(n1760), mab-5(e1239),andunc-3(n3435)are annotated as(-)and the hypomorphicunc-3alleleot837 [unc-3::mNG::AID]as(hypo). The identity of individual motor neurons is annotated. White arrowheads indicate MN nuclei because thecho-1reporter is localized to the nucleus (H2B).mChOptisignal is shown in white for better contrast. Left image: anterior to the vulva, Right image: posterior to the vulva.cQuantification of the number of motor neurons expressingcho-1in panel (b).n= 16–23 animals.dandeQuantification of the number of motor neurons (that control locomotion) expressingunc-17(endogenous reporterot907[UNC-17::mKate]) andace-2(fosmid-based reporterotEx4432[ace-2::GFP]) in multiple genetic backgrounds at L4 stage.n= 16–25 animals. For quantifications inc–e, box and whisker plots were used with the presentation of all data points. Unpairedt-test (two-sided) with Welch’s correction was performed andp-values were annotated. Box boundaries indicate the 25th and 75th percentile. The limits indicate minima and maxima values, whereas center values (mean) are highlighted in red.fSchematic summarizing our findings in cholinergic motor neurons that control locomotion. Source data are provided as a Source data file. Scale bar: 5 μm. Hox and other subfamilies of homeodomain proteins act as terminal selectors Homeodomain proteins are defined by a 60 amino acid motif (homeodomain) that directly contacts DNA [56] . Based on sequence similarities and/or the presence of other domains, several subfamilies of homeodomain proteins (e.g., HOX, LIM, POU, PRD) have been identified in every animal genome. In C. elegans , accumulating evidence suggests that members of LIM, POU, and PRD subfamilies can function as terminal selectors in specific neuron types [35] , [57] . Here, we show that members of the HOX subfamily can act as terminal selectors in cholinergic MNs. A synthesis of our findings and previous studies on LIM, POU, and PRD proteins reveals an overarching theme: a single transcription factor family, the homeodomain proteins, is broadly used in the C. elegans nervous system to control neuronal identity by acting as terminal selectors. Supporting the evolutionary conservation of this theme, a number of LIM and POU homeodomain transcription factors can function as terminal selectors in the mouse nervous system [9] , [10] , [58] , [59] , [60] . Hox proteins cooperate with the terminal selector UNC-3 (Collier/Ebf) to control motor neuron cholinergic identity Besides NT identity, terminal selectors are known to control additional neuron type-specific features of terminal differentiation, such as the expression of ion channels, neuropeptides, NT receptors, and cell adhesion molecules [46] , [48] . We find this to be the case for LIN-39. In sex-specific MNs that control egg laying, LIN-39 is required for continuous expression of ACh pathway genes and additional terminal differentiation markers (e.g., glr-5/GluR, ida-1/PTPRN ). Similarly, in MNs necessary for locomotion, LIN-39 controls ACh pathway genes (this study) and a handful of terminal differentiation markers (e.g., del-1 /sodium channel SCNN1, slo-2 /potassium–sodium-activated channel KCNT) [26] , [36] . But how can the same Hox protein (LIN-39) operate as a terminal selector in two different types of MNs? Our findings support the idea of LIN-39 cooperating with distinct transcription factors in different MN types. In MNs that control locomotion, LIN-39 synergizes with MAB-5 and UNC-3; the latter is known to function as a terminal selector in these neurons [14] . Mechanistically, LIN-39 and UNC-3 control the same ACh pathway genes by recognizing distinct binding sites. However, whether LIN-39 and UNC-3 are being recruited to these sites in an additive or cooperative manner remains unresolved. In MNs that control egg-laying [61] , UNC-3 is not present [14] . HLH-3 (bHLH protein of Achaete-Scute family) and LIN-11 (LIM homeodomain protein) are expressed in VC neurons [62] , [63] , constituting putative LIN-39 collaborators for the control of cholinergic identity in VC. Hox and UNC-3 in a positive feed-forward loop (FFL): a form of redundancy engineering to ensure robust expression of cholinergic identity genes Complex gene regulatory networks are composed of simple gene circuits called “network motifs” [64] . One of the most widely used motifs is the feed-forward loop (FFL), where transcription factor X activates a second transcription factor Y, and both activate their shared target gene Z (Fig. 5j ). Our findings uncovered a FFL in cholinergic MNs, where a Hox protein (LIN-39) activates UNC-3, and both activate their shared targets (ACh pathway genes) (Fig. 5j ). FFLs have been described in transcriptional networks across species [64] , [65] , [66] . Based on systems biology classifications, there are 8 different types of FFLs—each characterized by the signs (“+” for activation, “–” for repression) of the transcriptional interactions within the motif. The FFL in MNs is coherent type 1 because all interactions are activating (Fig. 5j ). Why is there a need for this type of FFL in C. elegans MNs? Computational models and studies in bacteria indicate that a coherent type 1 FFL can ensure robust gene expression against perturbations through a process called “sign-sensitive delay” [66] , [67] , [68] . That is, a perturbation can decrease the levels of transcription factor X (LIN-39), but Z (ACh pathway genes) responds only at a delay once X levels decrease. The delay is due to the presence of Y (UNC-3). After X is decreased, it takes time for Y levels to decrease (depending on the degradation rate of Y) to a level insufficient to activate Z. Hence, the coherent type 1 FFL can be viewed as a form of redundancy engineering (or filter) to protect the shared target genes (Z) from fluctuations in the input (transcription factor X). Based on computational modeling and functional studies in bacteria [66] , [67] , [68] , we propose that, in our system, LIN-39 (X) and UNC-3 (Y) operate in a coherent type 1 FFL to maintain robust expression levels of ACh pathway genes in MNs throughout life (Fig. 5j ). Lastly, we note that coherent and incoherent FFLs can serve various functions in the developing nervous system. For example, they can act as developmental timers (by allowing a given transcription factor to control different genes at successive developmental stages) [69] , [70] , [71] , or as means to generate neuronal subtype diversity [72] , [73] . The FFL we identified in C. elegans MNs forms the backbone of a transcriptional network, but it does not function in isolation. Rather, it is embedded within at least two additional loops: (a) a positive feedback loop that activates LIN-39 expression through transcriptional autoregulation, and (b) negative feedback provided by UNC-3 to reduce LIN-39 expression (Fig. 7g ). The significance of both is discussed below. Consistent with our observations on Hox (LIN-39, MAB-5) and unc-3 , two other C. elegans Hox proteins (CEH-13, EGL-5) control the transcription of another terminal selector ( mec-3 ) in peripheral touch receptor neurons [74] . Although a FFL was not identified in that cellular context, the findings on mec-3 and unc-3 (this study) strongly suggest that Hox-mediated transcriptional control of terminal selectors may be a broadly applicable strategy to ensure the robustness of gene expression in post-mitotic neurons. A two-component design principle for homeostatic control of Hox gene expression in motor neurons Mechanisms for the initiation of Hox gene expression are well-studied. 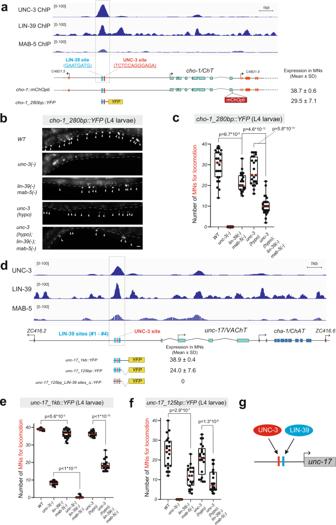Fig. 4: LIN-39 and UNC-3 act directly to activate the expression of ACh pathway genes. aGene locus ofcho-1with ChIP-seq tracks for UNC-3, LIN-39, and MAB-5. Molecular nature ofcho-1reporter genecho-1::mChOptiandcho-1_280bp::YFPis shown. Total number of MNs expressing each reporter is indicated in the format of mean ± standard derivation (SD). Within a 280 bpcis-regulatory region (gray dashed line), an UNC-3 site and a predicted LIN-39 site are highlighted in red and blue, respectively. MAB-5 binding sites are not shown because they are not well-defined.bRepresentative images ofcho-1_280bp::YFPexpression at L4 inWT, unc-3(n3435), lin-39(n1760) mab-5(e1239), unc-3(hypo),andunc-3(hypo); lin-39(n1760); mab-5(e1239)animals. Arrowheads indicate MN nuclei becausecho-1_280bp::YFPhas a nuclear localization signal (NLS). YFP signal is shown in white for better contrast. Dashed white lines indicate the boundary of the intestine, which is auto-fluorescent in the green channel.cQuantification of the number of motor neurons expressingcho-1 reporterin panel (b).n= 18–27 animals.d. Gene locus ofunc-17with ChIP-seq tracks for UNC-3, LIN-39, and MAB-5. Expression in motor neurons is quantified forunc-17reporter genes (unc-17_1kb::YFPandunc-17_125bp::YFP),as well as its mutated version with LIN-39 site deletions. Within a 125 bpcis-regulatory region framed by the gray dashed line, a UNC-3 site and 4 predicted LIN-39 sites are highlighted in red and blue, respectively.eandfQuantification of the number of motor neurons at L4 expressing theunc-17_1kb::YFP(e) andunc-17_125bp::YFP(f) reporters inWT, unc-3(n3435), lin-39(n1760); mab-5(e1239), unc-3(n3435), lin-39(n1760); mab-5(e1239), unc-3(hypo), and unc-3(hypo); lin-39(n1760); mab-5(e1239)animals. For all quantifications, box and whisker plots were used with the presentation of all data points. Box boundaries indicate the 25th and 75th percentile. The limits indicate minima and maxima values, whereas center values (mean) are highlighted in red. Unpairedt-test (two-sided) with Welch’s correction was performed and p-values were annotated.n= 15–26 animals.gSchematic ofunc-17regulation by UNC-3, LIN-39, and MAB-5. Red and blue rectangles indicate the binding sites of UNC-3 and LIN-39, respectively. Source data are provided as a Source data file. Scale bar: 5 μm. It is known, for example, that during embryonic patterning, Polycomb Group (PcG) and trithorax Group (trxG) genes determine the levels and spatial expression of Hox genes [75] , [76] , [77] , [78] , [79] . It is also known that, during early nervous system development, morphogenetic gradients initially establish Hox gene expression, and this is further refined via Hox cross-regulatory interactions [22] , [80] . However, the mechanisms that maintain Hox gene expression in post-mitotic neurons during later developmental and post-embryonic stages remain unknown. Our constitutive (genetic null alleles) and temporally controlled (AID system) approaches combined with mutagenesis of Hox binding sites within the endogenous lin-39 locus strongly suggest that LIN-39 maintains its own expression in MNs through transcriptional autoregulation (Fig. 6i ). Subsequently, LIN-39 is required to maintain the expression of ACh pathway genes by operating at the top of a coherent FFL (Fig. 6j ). However, the lin-39 expression levels are critical: low levels lead to a failure to maintain ACh pathway gene expression (Figs. 1 and 2 ), whereas high levels of LIN-39 in cholinergic MNs cause locomotion defects and “mixed neuronal identity”, i.e., genes normally expressed in GABA neurons became ectopically expressed in cholinergic MNs [36] . We found that lin-39 expression in MNs is under homeostatic control. The terminal selector UNC-3 prevents high levels of lin-39 expression, thereby counterbalancing the positive effect of the transcriptional autoregulation of lin-39 . From the perspective of Hox binding site affinity [81] , [82] , this mechanism may enable LIN-39 (when present at optimal levels) to bind at high-affinity sites in the cis -regulatory region of ACh pathway genes. The negative UNC-3 feedback prevents high levels of LIN-39, potentially avoiding LIN-39 binding to low-affinity sites in the cis -regulatory region of alternative (e.g., GABA) identity genes. Altogether, we identified a two-component design principle (positive feedback of LIN-39 to itself, negative feedback from the terminal selector UNC-3) for the homeostatic control of Hox gene expression in motor neurons. These two components are embedded in a coherent FFL, which we propose to be necessary for the maintenance of NT identity (Fig. 7g ). Because Hox genes are continuously expressed in the adult fly, mouse, and human nervous systems, the gene regulatory architecture described here for the control of NT identity may constitute a broadly applicable principle. 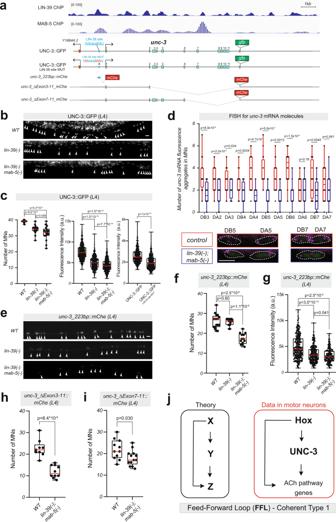Fig. 5: LIN-39 and MAB-5 controlunc-3expression levels. aChIP-seq tracks for LIN-39 and MAB-5 onunc-3locus. Molecular nature of endogenousunc-3reporters (UNC-3::GFP and UNC-3::GFPLIN-39 site MUT) and transgenicunc-3reporters(unc-3_223bp::mChe, unc-3_ΔExon3-11_mChe,unc-3_ΔExon7-11_mChe).bRepresentative images of L4 animals carrying the endogenousunc-3::gfpreporter inWT, lin-39(n1760), andlin-39(n1760); mab-5(e1239)backgrounds.cQuantification of MN number (left graph,n= 19–22 animals) or fluorescence intensity (middle graph,n= 595 neurons) of UNC-3::GFP in WT, lin-39(n1760), and lin-39(n1760); mab-5(e1239)backgrounds. Right graph: Quantification of fluorescent GFP intensity in MNs of animals carrying theUNC-3::GFP andUNC-3::GFPLIN-39 site MUTendogenous reporters.n= 682 neurons.dQuantification of the number ofunc-3mRNA fluorescence aggregates in individual cholinergic MNs. Single-molecule mRNA FISH forunc-3was performed in WT andlin-39(n1760); mab-5(e1239)animals at L1. For all quantifications, box and whisker plots were used; all data points shown. Unpairedt-test with Welch’s correction was performed andp-values were annotated.n= 22 animals. Representative images of DB5, DA5, DB7, and DA7 neurons. WT (colored red) versus mutant (in blue) for quantification. Magenta: signal from Quasar 670 probe forunc-3mRNA, Green:unc-17::gfpreporter for cholinergic motor neurons.eRepresentative images ofunc-3_223bp::mCheexpression in L4 hermaphrodites inWT, lin-39(n1760), andlin-39(n1760); mab-5(e1239).fandgQuantification of MN numbers (f,n= 13–17 animals) or fluorescence intensity (g,n= 176 neurons) ofunc-3_223bp::mChein panel (e). For fluorescence intensity quantifications, single neurons expressing the mCherry reporters are plotted as individual data points.n> 600. In panelg,n> 200 neurons.handiQuantification of the number of MNs expressing theunc-3_ΔExon3-11_mChe(h), andunc-3_ΔExon7-11_mChe(i)in WT and lin-39(n1760); mab-5(e1239)mutant animals.n= 10 animals. For all quantifications, box and whisker plots were used; all data points were presented. Box boundaries indicate the 25th and 75th percentile. The limits indicate minima and maxima values, whereas center values (mean) are highlighted in red. Unpairedt-test (two-sided) with Welch’s correction was performed.jSchematic model of a coherent feed-forward loop (FFL) for the control of cholinergic identity. Source data are provided as a Source data file. Scale bars: 5 μm. C. elegans strains Worms were grown at 15, 20, or 25 °C on nematode growth media (NGM) plates seeded with bacteria ( E. coli OP50) as food source [83] . Mutant alleles used in this study: unc-3 (n3435) X, lin-39 (n1760) III, mab-5 (e1239) III, ced-3 (n1286) IV . CRISPR-generated alleles: unc-3 (ot837 [unc-3::mNG::3xFLAG::AID]) X, lin-39 (kas9 [lin-39::mNG::3xFLAG::AID]) III . All reporter strains used in this study are shown in Supplementary Data 1 . Generation of transgenic reporter animals Reporter gene fusions for cis -regulatory analysis were made using either PCR fusion [84] or Gibson Assembly Cloning Kit (NEB #5510S). Targeted DNA fragments were fused (ligated) to the tagrfp -coding sequence, which was followed by unc-54 3’ UTR . Mutations or deletions of LIN-39-binding sites were introduced via PCR mutagenesis. The product DNA fragments were either injected into young adult pha-1(e2123) hermaphrodites at 50 ng/µl using pha-1 (pBX plasmid) as co-injection marker (50 ng/µl) and further selected for survival, or injected into young adult N2 hermaphrodites at 50 ng/µl (plus 50 ng/µl pBX plasmid) using myo-2::gfp as co-injection marker (3 ng/µl) and further selected for GFP signal. Targeted genome engineering CRISPR/Cas9 genome editing was employed to generate: (a) PHX2477 strain carrying the lin-39(syb2477 [lin-39_site1-11_MUT::mNG::3xFLAG::AID]) III allele, and (b) PHX5816 strain carrying the unc-3(syb5816 [unc-3_LIN-39 site_MUT_GFP]) X allele. Gene editing was performed by SunyBiotech. Temporally controlled protein degradation AID-tagged proteins are conditionally degraded when exposed to auxin in the presence of TIR1 [37] . Animals carrying auxin-inducible alleles of lin-39 (kas9 [lin-39::mNG::AID]) were crossed with ieSi57 animals that express TIR1 ubiquitously or with otTi28 animals that express TIR-1 pan-neuronally. Auxin (indole-3-acetic acid [IAA], Catalog number A10556, Alfa Aesar) was dissolved in ethanol (EtOH) to prepare 400 mM stock solutions which were stored at 4 °C for up to one month. NGM agar plates were poured with auxin or ethanol added to a final concentration of 4 mM and allowed to dry overnight at room temperature. Plates were seeded with OP50 bacteria. To induce protein degradation, worms of the experimental strains were transferred onto auxin-coated plates and kept at 25 °C. As a control, worms were transferred onto EtOH-coated plates instead. Auxin solutions, auxin-coated plates, and experimental plates were shielded from light. Single molecule RNA in situ hybridization (sm RNA-FISH) Egg preparation was performed before harvesting the synchronized L1 worms. Next, worms were fixed with 4% paraformaldehyde (PFA), washed twice with PBS, and permeabilized with 70% ethanol at 4 °C overnight. Then, samples were hybridized with diluted mRNA probes (Stellaris; unc-3 : unc-3 best Quasar 670 (SMF-1065-5); lin-39 : lin-39 best Quasar 670 (SMF-1065-5)) in hybridization buffer (Stellaris#174; RNA FISH hybridization buffer (SMF-HB1-10)) following manufacturing protocols. Finally, samples were stained with DAPI, washed, and equilibrated with GLOX buffer. Worms were imaged at a fluorescence microscope (Zeiss, Axio Imager.Z2). Real-time PCR assay for unc-3 and lin-39 expression level analysis Synchronized L4 stage C. elegans animals were collected from different genotypes (see figure legends), and mRNA was extracted. cDNA library was prepared using the Superscript first strand cDNA synthesis kit (Invitrogen #11904-018). RT-PCR TaqMan assays for the genes unc-3 (assay ID: Ce02402729_g1), lin-39 (assay ID: Ce02406896_m1), and pmp-3 (Ce02485188_m1) were performed, and the expression level of unc-3 and lin-39 were determined in each genotype after normalizing to the expression of the housekeeping gene pmp-3 . Microscopy Worms were anesthetized using 100 mM of sodium azide (NaN 3 ) and mounted on a 4% agarose pad on glass slides. Images were taken using an automated fluorescence microscope (Zeiss, Axio Imager.Z2). Acquisition of several Z-stack images (each ~1 µm thick) was taken with Zeiss Axiocam 503 mono using the ZEN software (Version 2.3.69.1000, Blue edition). Representative images are shown following max-projection of 1–8 µm Z-stacks using the maximum intensity projection type. Image reconstruction was performed using Image J software [85] . Motor neuron identification Motor neurons were identified based on a combination of the following factors: (i) co-localization with fluorescent markers with known expression pattern, (ii) invariant cell body position along the ventral nerve cord, or relative to other MN subtypes, (iii) MN birth order, and (iv) number of MNs that belong to each subtype. Bioinformatic analysis To predict the UNC-3-binding site (COE motif) in the cis -regulatory region of target genes, we used the MatInspector program from Genomatix [86] . The position weight matrix (PWM) for the LIN-39-binding site is cataloged in the CIS-BP (Catalog of Inferred Sequence Binding Preferences database) [87] . To identify putative LIN-39 sites, we used FIMO (Find Individual Motif Occurrences) [88] , which is one of the motif-based sequence analysis tools of multiple expectation maximization for motif elicitation (MEME) bioinformatics suites ( http://meme-suite.org/ ). The p -value threshold for the analysis of LIN-39 target genes was set at p < 0.001 for unc-17 and cho-1 , and at p < 0.01 for lin-39 . Fluorescence intensity (FI) quantification To quantify FI of individual MNs in the VNC, images of worms from different genetic backgrounds were taken with identical parameters through full-thickness Z-stacks that cover the entire cell body. Image stacks were then processed and quantified for FI via FIJI. The focal plane in Z-stacks that has the brightest FI was selected for quantification to minimize background signals. Cell outline was manually selected, and FIJI was used to quantify the FI and area to get the mean value for FI. After quantifying the FI of all MNs of interest, representative average image background FI was quantified and subtracted from the individual MN FI quantifications to get the mean FI in arbitrary units (a.u.). Statistical analysis and reproducibility For quantification, box and whisker plots were adopted to represent the quartiles in graph. The box includes data points from the first to the third quartile value with the horizontal line in box representing the mean value. Upper and lower limits indicate the max and min, respectively. Unpaired t -test with Welch’s correction was performed and p -values were annotated. Visualization of data and p -value calculation were performed via GraphPad Prism Version 9.2.0 (283). Each experiment was repeated twice. 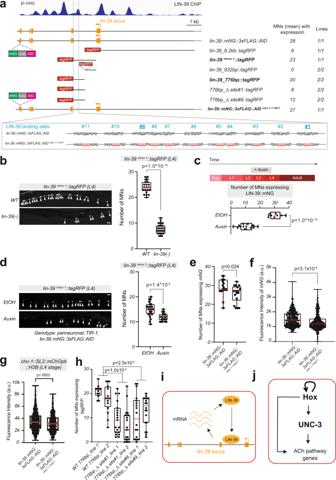Fig. 6: Transcriptional autoregulation oflin-39in motor neurons. aChIP-seq tracks for LIN-39 onlin-39locus. Molecular nature of endogenouslin-39reporters (lin-39::mNG::3xFLAG::AIDandlin-39::mNG::3xFLAG::AIDsites1-11MUT)and transgeniclin-39reporters(lin-39_6.2kb::tagRFP,lin-39intron1::tagRFP, lin-39_832bp::tagRFP,lin-39_776bp::tagRFP,776bp_Δsite#1::tagRFP,776bp_Δsite#9::tagRFP). The mean value of MNs that express each reporter is indicated on the right. The precise location of the 11 predicted LIN-39 binding sites is shown, and their mutated version.bRepresentative images and quantification of the number of MNs expressinglin-39intron1::tagRFPinWTandlin-39(n1760)mutants at L4.n= 21–30 animals.cDepletion of LIN-39::mNG::3xFLAG::AID upon auxin. Worms expressing thelin-39::mNG::3xFLAG::AIDtogether with TIR protein in all neurons (driven by pan-neuronal promoterotti28) were grown on normal OP50 plates until L2 stage and then transferred to plates containing either auxin or EtOH (as control). Animals were imaged at L4. Quantification of LIN-39::mNG::3xFLAG::AID expression in motor neurons upon Auxin or EtOH treatment.n= 8–15 animals.dRepresentative images and quantification of the number of MNs expressinglin-39intron1::tagRFPtreated with EtOH or auxin.n= 26-28 animals.eandfQuantification (L4 stage) of the number of MNs expressingmNG(e,n= 18–19 animals) or the fluorescence intensity (f,n= 459 neurons) ofmNGin animals carrying thelin-39::mNG::3xFLAG::AIDandlin-39::mNG::3xFLAG::AIDsites1-11MUTalleles. In panelf, single neurons expressingmNGare plotted as individual data points.n> 400 cells. a.u. arbitrary units.gQuantification of fluorescent intensity ofcho-1::SL2::mChOpti::H2Bexpression in MNs oflin-39::mNG::3xFLAG::AIDorlin-39::mNG::3xFLAG::AIDsites1-11MUTanimals (L4 stage).hQuantification of the number of MNs expressing thelin-39_776bp::tagRFPreporter (intact and mutated version with LIN-39 site#1 or #9 mutated). Two independent transgenic lines for each version of the reporter were used.n= 12–21 animals. For all quantifications, box and whisker plots were used; all data points were presented. Box boundaries indicate the 25th and 75th percentile. The limits indicate minima and maxima values, whereas center values (mean) are highlighted in red. Unpairedt-test (two-sided) with Welch’s correction was performed.n> 15 animals.iSchematic model oflin-39transcriptional autoregulation.jSchematic model showing the autoregulation oflin-39embedded at the top of a coherent FFL. Source data are provided as a Source data file. Scale bars: 5 μm. 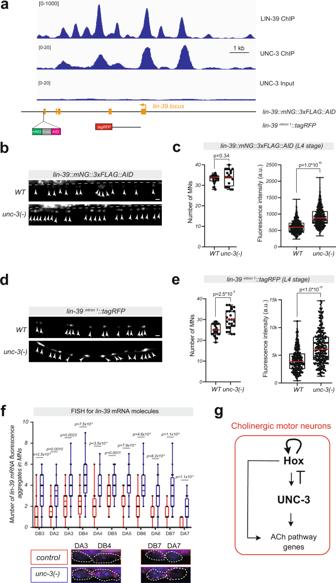Fig. 7: UNC-3 (Collier/Ebf) prevents high levels oflin-39expression. aGene locus oflin-39with ChIP-seq tracks for UNC-3 and LIN-39. Molecular nature oflin-39reporter genelin-39::mNG::3xFLAG::AIDandlin-39intron1::tagRFPis shown.bandcRepresentative images (b) and quantifications (c) of the number of MNs (n= 20 animals) expressinglin-39::mNG::3xFLAG::AIDand the fluorescence intensity (n= 660 neurons) inWTandunc-3(n3435)animals at L4.dandeRepresentative images (d) and quantifications (e) of the number (n= 23 animals) and the fluorescence intensity (n= 264 neurons) of MNs expressinglin-39intron1::tagRFPinWTversusunc-3(n3435)animals at L4. In panelscande, single neurons expressing the indicated reporter gene are evaluated for fluorescence intensity and plotted as individual data points in the graph.n> 600 neurons. a.u. arbitrary unit.fQuantification of the number oflin-39mRNA fluorescence aggregates in individual cholinergic MNs. Single-molecule mRNA FISH forlin-39 (using a Quasar 670 fluorescent probe) was performed in WT andunc-3(n3435)animals at L1 (n= 20 animals). For all quantifications, box and whisker plots were used with the presentation of all data points. Box boundaries indicate the 25th and 75th percentile. The limits indicate minima and maxima values, whereas center values (mean) are highlighted in red. Unpairedt-test (two-sided) with Welch’s correction was performed andp-values were annotated.n> 20 animals. Representative images of DA3, DB4, DB7, and DA7 are shown. WT data is colored red versus mutant in blue for quantification. Images are shown in merged channels. Magenta: signal from Quasar 670 probe forlin-39mRNA, Blue: DAPI for nuclei staining.gSchematic model of the gene regulatory network for maintenance of cholinergic identity inC. elegansmotor neurons. Source data are provided as a Source data file. Scale bars: 5 μm. Reporting summary Further information on research design is available in the Nature Research Reporting Summary linked to this article.